Fluid flow and interlinked feedback loops establish left–right asymmetric decay ofCerl2mRNA Breaking of left–right symmetry in mouse embryos requires fluid flow at the node, but the precise action of the flow has remained unknown. Here we show that the left–right asymmetry of Cerl2 expression around the node, a target of the flow, is determined post-transcriptionally by decay of Cerl2 mRNA in a manner dependent on its 3′ untranslated region. Cerl2 mRNA is absent specifically from the apical region of crown cells on the left side of the node. Preferential decay of Cerl2 mRNA on the left is initiated by the leftward flow and further enhanced by the operation of Wnt-Cerl2 interlinked feedback loops, in which Wnt3 upregulates Wnt3 expression and promotes Cerl2 mRNA decay, whereas Cerl2 promotes Wnt degradation. Mathematical modelling and experimental data suggest that these feedback loops behave as a bistable switch that can amplify in a noise-resistant manner a small bias conferred by fluid flow. During development of the mouse embryo, unidirectional fluid flow (nodal flow) breaks left–right (L–R) symmetry at the embryonic node [1] . Nodal flow is generated by clockwise rotation of multiple cilia that are positioned at the posterior side of node cells by the planar cell polarity pathway [2] , [3] , [4] , and it promotes asymmetric gene expression around the node. The first gene to show asymmetric expression around the node is that for Cerl2 (Cerberus-like protein 2), which is expressed in perinodal crown cells in a L<R manner and has a key role in L–R determination as an inhibitor of the protein Nodal [5] , [6] . The activity of Nodal is repressed asymmetrically around the node by Cerl2, and the resulting L>R asymmetric pattern of Nodal activity is transmitted to the lateral plate mesoderm (LPM) [6] , [7] . Mutant mice lacking Cerl2 expression thus manifest randomized expression of Nodal in LPM [5] . In the LPM of wild-type embryos, the asymmetric activity of Nodal derived from the node is amplified by a self-enhancement and lateral-inhibition (SELI) system, resulting in an exclusively left-sided pattern of Nodal expression [8] . However, it remains unknown how asymmetric expression of Cerl2 around the node is established by nodal flow, which fluctuates with time and therefore may provide an unstable signal. If the flow-derived signal indeed fluctuates, how is the initial ambiguous or subtle asymmetry converted to robust asymmetry of gene expression? Many processes that take place in a cell or in a multicellular organism show stochastic fluctuation. For example, gene expression manifests endogenous noise that originates from the transcription and translation steps [9] , [10] , [11] . In addition, gene expression is affected by exogenous noise [9] , [10] . The development of an embryo consisting of multiple cells must thus proceed in the presence of such noise. How stochastic fluctuation is absorbed in living organisms is largely unknown, but theoretical modelling and experiments with unicellular organisms have suggested that feedback loops in genetic circuits have an important role in noise reduction [12] , [13] . We have now examined how L<R asymmetry of Cerl2 expression is established in perinodal crown cells of the mouse embryo. Genetic and embryonic manipulations as well as mathematical modelling revealed that robust asymmetry in the distribution of Cerl2 mRNA is generated by preferential decay of the mRNA on the left side, which is initiated by nodal flow and subsequently promoted by the operation of Wnt-Cerl2 interlinked feedback loops. This mechanism ensures that asymmetry of Cerl2 expression is established with high accuracy in a noise-resistant manner. L–R asymmetric distribution of Cerl2 mRNA via its 3′-UTR Cerl2 mRNA exhibits a dynamic L–R asymmetric pattern of distribution around the node of the mouse embryo [5] . Fluorescence in situ hybridization (FISH) with an exon probe reveals a L=R pattern for Cerl2 mRNA at the early headfold stage but a R>L pattern at the late headfold stage. The R>L asymmetry of Cerl2 mRNA becomes more obvious at the two pairs of somites stage (2 pss) ( Fig. 1a ). Examination of Cerl2 expression with an intron probe, however, revealed no obvious difference in the abundance of Cerl2 mRNA between the left and right sides of the node at 2 or 3 pss ( Fig. 1b , Supplementary Fig. S1 ), suggesting that L–R asymmetry of Cerl2 mRNA is determined mainly at a post-transcriptional level (as a few embryos shown in Fig. 1c show R>L pattern, transcriptional regulation may also have a minor role). This conclusion was further supported by analysis of the effects of actinomycin D, a specific inhibitor of RNA polymerase. For mouse embryos cultured in the presence of actinomycin D from 1 to 3 pss, the intron probe failed to detect Cerl2 mRNA (3/3 embryos) ( Fig. 1d ), whereas the exon probe still revealed R>L asymmetry of Cerl2 mRNA (3/3 embryos) ( Fig. 1f ). We next examined the expression of lacZ from the Cerl2 lacZ allele, in which the second exon of Cerl2 has been replaced with the coding sequence for β-galactosidase and the polyadenylation signal sequence of SV40 (ref. 5 ). The distribution of lacZ mRNA in Cerl2 lacZ/lacZ embryos did not show obvious L–R asymmetry at 3 pss ( Fig. 1h ). Similarly, a symmetric distribution of lacZ mRNA was apparent at this stage in embryos harbouring a Cerl2 ( lacZ ) BAC (bacterial artificial chromosome) transgene ( Fig. 1i ), in which lacZ and the SV40 polyadenylation signal sequence are added to Cerl2 in the same manner as for the Cerl2 lacZ allele. 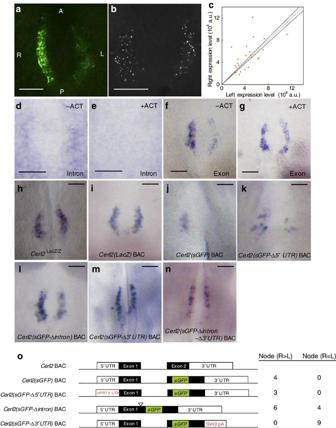Figure 1: The R>L asymmetric distribution ofCerl2mRNA is generated post-transcriptionally via its 3′-UTR. (a) Whole-mount FISH analysis ofCerl2mRNA with an exon probe in the node region of a mouse embryo at 2 pss. (b) Whole-mount FISH analysis as in (a) with aCerl2intron probe. (c) Quantitative FISH analysis ofCerl2mRNA with an intron probe. Each data point represents the sum of the abundance ofCerl2mRNA per embryo (a.u., arbitrary units) determined for crown cells on the left or right side of the node for an individual embryo at 1–3 pss. Dashed line indicates 5% fluctuated line from centre line (L=R). For each amount ofCerl2RNA inside the nucleus, see alsoSupplementary Fig. S4. (d–g) Whole-mountin situhybridization (WISH) analysis ofCerl2mRNA with an intron probe (d,e) or an exon probe (f,g) in embryos cultured without (d,f) or with (e,g) 1 μg μl−1actinomycin D (ACT) from 1 to 3 pss. (h) Whole-mount WISH analysis oflacZmRNA in aCerl2lacZ/lacZembryo at 3 pss. (i) WISH analysis oflacZmRNA in aCerl2(lacZ) BAC transgenic embryo at 3 pss. (j–n) WISH analysis ofCerl2(sGFP) mRNA with ansGFPprobe in embryos harbouring the indicated BAC transgenes at 3 pss. Scale bars: 50 μm. (o) Schematic representation of BAC transgenes and summary of the results obtained for the distribution ofCerl2(sGFP) BAC transcripts around the node. Figure 1: The R>L asymmetric distribution of Cerl2 mRNA is generated post-transcriptionally via its 3′-UTR. ( a ) Whole-mount FISH analysis of Cerl2 mRNA with an exon probe in the node region of a mouse embryo at 2 pss. ( b ) Whole-mount FISH analysis as in ( a ) with a Cerl2 intron probe. ( c ) Quantitative FISH analysis of Cerl2 mRNA with an intron probe. Each data point represents the sum of the abundance of Cerl2 mRNA per embryo (a.u., arbitrary units) determined for crown cells on the left or right side of the node for an individual embryo at 1–3 pss. Dashed line indicates 5% fluctuated line from centre line (L=R). For each amount of Cerl2 RNA inside the nucleus, see also Supplementary Fig. S4 . ( d – g ) Whole-mount in situ hybridization (WISH) analysis of Cerl2 mRNA with an intron probe ( d , e ) or an exon probe ( f , g ) in embryos cultured without ( d , f ) or with ( e , g ) 1 μg μl −1 actinomycin D (ACT) from 1 to 3 pss. ( h ) Whole-mount WISH analysis of lacZ mRNA in a Cerl2 lacZ/lacZ embryo at 3 pss. ( i ) WISH analysis of lacZ mRNA in a Cerl2 ( lacZ ) BAC transgenic embryo at 3 pss. ( j – n ) WISH analysis of Cerl2 ( sGFP ) mRNA with an sGFP probe in embryos harbouring the indicated BAC transgenes at 3 pss. Scale bars: 50 μm. ( o ) Schematic representation of BAC transgenes and summary of the results obtained for the distribution of Cerl2 ( sGFP ) BAC transcripts around the node. Full size image To determine which region of Cerl2 is responsible for the R>L asymmetry of Cerl2 mRNA, we generated the Cerl2 ( sGFP ) BAC transgene, in which a 300-bp portion of the coding sequence for enhanced green fluorescence protein ( sGFP ) is inserted into exon 2 of Cerl2 . This transgene generates Cerl2 mRNA with an sGFP tag but does not produce functional Cerl2 protein. Embryos harbouring the Cerl2 ( sGFP ) BAC transgene showed R>L asymmetry of Cerl2 mRNA, as detected with a GFP antisense probe, at 2–3 pss ( Fig. 1j ). We then deleted or replaced various regions (5′-UTR, intron, or 3′-UTR) of the Cerl2 ( sGFP ) BAC transgene. Cerl2 ( sGFP- Δ 5 ′- UTR ), in which the 5′-UTR of Cerl2 is replaced by the 5′-UTR of the hypoxanthine-guanine phosphoribosyltransferase gene ( Hprt ), showed R>L asymmetry of Cerl2 ( sGFP ) mRNA ( Fig. 1k ), similar to that observed with the Cerl2 ( sGFP ) BAC transgene. Cerl2 ( sGFP- Δ intron ), which lacks the Cerl2 intron, showed R>L expression (6/10 embryos) or bilaterally equal expression (4/10 embryos) ( Fig. 1l ). In contrast, both Cerl2 ( sGFP- Δ 3 ′ UTR ), in which the 3′-UTR of Cerl2 is replaced by the 3′-UTR of SV40, and Cerl2 ( sGFP- Δ intron Δ 3 ′- UTR ) showed a symmetric distribution of Cerl2 ( sGFP ) mRNA ( Fig. 1m–o ). These results thus suggested that the L–R asymmetry of Cerl2 mRNA is determined post-transcriptionally mainly via its 3′-UTR. Subcellular localization of Cerl2 mRNA We examined the subcellular distribution of Cerl2 mRNA in crown cells at the node by whole-mount FISH analysis. Although Cerl2 mRNA was detected in both the apical and basal regions of crown cells on the right side of the node at 3 pss, it was absent or rarely detected in the apical region of crown cells on the left side ( Fig. 2a ). Statistical analysis of multiple embryos at 1, 2 and 3 pss confirmed that apical localization of Cerl2 mRNA takes place preferentially on the right side ( Supplementary Fig. S2 ). In iv/iv mutant embryos, which lack nodal flow, the distribution of Cerl2 mRNA was randomized; it was either absent in the apical region of left crown cells ( Fig. 2c ) or absent in the apical region on right ( Fig. 2e ). Furthermore, embryos harbouring the Cerl2 ( sGFP- Δ 3 ′ -UTR ) BAC transgene manifested neither L–R asymmetry nor apicobasal polarity of Cerl2 ( sGFP ) mRNA ( Fig. 2g ). These results thus suggested that Cerl2 mRNA is degraded in the apical region of crown cells on the left side of the node in a manner dependent on its 3′-UTR and in response to nodal flow. 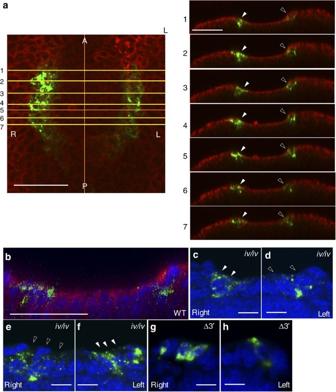Figure 2: Subcellular localization ofCerl2mRNA in crown cells. (a) Whole-mount FISH analysis ofCerl2mRNA with an exon probe (green fluorescence) in a mouse embryo at 3 pss. The embryo was also stained with DiI (red fluorescence) to reveal the apical membrane of crown cells. Only the node region is shown. Sections along the anteroposterior axis shown in the left panel were randomly selected and are shown in sequence in the right panel.Cerl2mRNA is present in the apical region of crown cells on the right side of the node (closed arrowheads) but not in that of left crown cells (open arrowheads). This is especially obvious in the posterior portion of the node, where nodal flow is efficient. (b) Transverse section of an embryo at 3 pss subjected to whole-mount FISH analysis ofCerl2mRNA with an exon probe (green) as well as to DiI staining (red) to reveal the apical surface. Nuclei were also stained with 4′,6-diamidino-2-phenylindole (DAPI, blue). (c–f)Cerl2mRNA localization iniv/ivmutant embryos determined as in (b). Two patterns of localization are shown in (c) and (d) and in (e) and (f). Closed and open arrowheads indicate the presence or absence, respectively, ofCerl2mRNA in the apical region of crown cells. (g,h)Cerl2-sGFPmRNA localization in an embryo harboring theCerl2(sGFP-Δ3′UTR) BAC transgene determined as in (b). Scale bars: 50 μm(a,b), Scale bars: 10 μm(c–h). Figure 2: Subcellular localization of Cerl2 mRNA in crown cells. ( a ) Whole-mount FISH analysis of Cerl2 mRNA with an exon probe (green fluorescence) in a mouse embryo at 3 pss. The embryo was also stained with DiI (red fluorescence) to reveal the apical membrane of crown cells. Only the node region is shown. Sections along the anteroposterior axis shown in the left panel were randomly selected and are shown in sequence in the right panel. Cerl2 mRNA is present in the apical region of crown cells on the right side of the node (closed arrowheads) but not in that of left crown cells (open arrowheads). This is especially obvious in the posterior portion of the node, where nodal flow is efficient. ( b ) Transverse section of an embryo at 3 pss subjected to whole-mount FISH analysis of Cerl2 mRNA with an exon probe (green) as well as to DiI staining (red) to reveal the apical surface. Nuclei were also stained with 4′,6-diamidino-2-phenylindole (DAPI, blue). ( c – f ) Cerl2 mRNA localization in iv / iv mutant embryos determined as in ( b ). Two patterns of localization are shown in ( c ) and ( d ) and in ( e ) and ( f ). Closed and open arrowheads indicate the presence or absence, respectively, of Cerl2 mRNA in the apical region of crown cells. ( g , h ) Cerl2-sGFP mRNA localization in an embryo harboring the Cerl2 ( sGFP- Δ 3 ′ UTR ) BAC transgene determined as in ( b ). Scale bars: 50 μm( a , b ), Scale bars: 10 μm( c – h ). Full size image Ambiguous L–R asymmetry of Cerl2 mRNA at early stages Although Cerl2 expression is dynamic in individual embryos, its level also varies among embryos at the same stage ( Supplementary Fig. S3 ). The amounts of Cerl2 and Nodal mRNAs in individual embryos at various stages were simultaneously and quantitatively determined by two-color FISH analysis ( Fig. 3a–e , Supplementary Fig. S4 ). The two mRNAs showed substantial variation in both their abundance and asymmetry among embryos at 1, 2 or 3 pss. Although the amount of Cerl2 mRNA relative to that of Nodal mRNA did not exhibit obvious L–R asymmetry at 1 pss, it showed marked L<R asymmetry at 3 pss (even though the level of Cerl2 expression still varied among individual embryos). 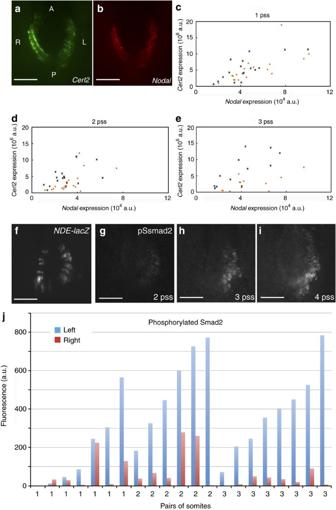Figure 3: Asymmetry ofCerl2mRNA is ambiguous in and varies among early-stage embryos. (a,b) Whole-mount FISH analysis ofCerl2mRNA with an exon probe (a) andNodalmRNA (b) in the same embryo at 1 pss. (c–e) Quantitative FISH analysis ofNodalandCerl2expression at 1 pss (c), 2 pss (d) or 3 pss (e). Each data point represents the abundance ofCerl2andNodalmRNAs on the right41or left (orange) side of the node in one embryo. (f) Immunofluorescence analysis of β-galactosidase in a 3-pss embryo harbouring theNDE-lacZtransgene, in whichlacZis controlled by the node-specific enhancer ofNodal. (g–i) Immunofluorescence staining of phosphorylated Smad2 (pSmad2) around the node at 2 pss (g), 3 pss (h) or 4 pss (i). (j) Quantitative analysis of pSmad2 immunostaining. Each pair of blue and red bars indicates the level of staining on the left and right sides, respectively, of the node of one embryo at the indicated stages. See alsoSupplementary Figs S2,S3. Scale bars, 50 μm. Figure 3: Asymmetry of Cerl2 mRNA is ambiguous in and varies among early-stage embryos. ( a , b ) Whole-mount FISH analysis of Cerl2 mRNA with an exon probe ( a ) and Nodal mRNA ( b ) in the same embryo at 1 pss. ( c – e ) Quantitative FISH analysis of Nodal and Cerl2 expression at 1 pss ( c ), 2 pss ( d ) or 3 pss ( e ). Each data point represents the abundance of Cerl2 and Nodal mRNAs on the right [41] or left (orange) side of the node in one embryo. ( f ) Immunofluorescence analysis of β-galactosidase in a 3-pss embryo harbouring the NDE-lacZ transgene, in which lacZ is controlled by the node-specific enhancer of Nodal . ( g – i ) Immunofluorescence staining of phosphorylated Smad2 (pSmad2) around the node at 2 pss ( g ), 3 pss ( h ) or 4 pss ( i ). ( j ) Quantitative analysis of pSmad2 immunostaining. Each pair of blue and red bars indicates the level of staining on the left and right sides, respectively, of the node of one embryo at the indicated stages. See also Supplementary Figs S2,S3 . Scale bars, 50 μm. Full size image We also determined the level of phosphorylated Smad2 (pSmad2) on each side of the node by quantitative immunofluorescence analysis ( Fig. 3g–j ). The level of pSmad2 would represent the net Nodal activity (the level of Nodal protein minus that of Cerl2). Whereas L–R asymmetry of pSmad2 was ambiguous in ~50% of embryos at 1 pss, L>R asymmetry was obvious in all embryos examined at 2, 3 or 4 pss, similar (but opposite) to the pattern observed for Cerl2 expression. Wnt signalling is required for robust asymmetry of Cerl2 mRNA To identify the mechanism responsible for establishment of the robust asymmetry of Cerl2 mRNA, we searched for other genes that might show asymmetric expression around the node. Among Wnt and BMP (bone morphogenetic protein) genes examined, Wnt3 was found to show such expression ( Fig. 4 ). Wnt3 expression begins to show subtle L>R asymmetry at 2 pss ( Fig. 4a ), after which expression on the left side gradually increases and the L>R asymmetry becomes more pronounced (1/2, 5/6, 4/4 and 4/4 embryos showed asymmetric expression at 2, 3, 4 and 5 pss, respectively) ( Fig. 4b–d ). The asymmetry of Wnt3 expression was confirmed by examination of embryos harbouring the Wnt3 ( mVenus ) BAC transgene, in which the coding sequence for membrane-localized Venus is intercalated into start site of Wnt3 . L>R asymmetry of mVenus expression became apparent at 4 pss and was more pronounced at 5 pss (0/2, 1/1, 2/2 and 4/4 embryos showed asymmetric expression at 2, 3, 4 or 5 pss, respectively) ( Fig. 4e–g ). 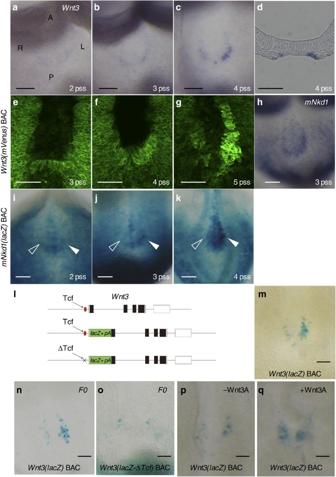Figure 4: Asymmetric expression ofWnt3and its regulation by Wnt signalling. (a–d) WISH analysis ofWnt3expression at 2 pss (a), 3 pss (b) and 4 pss (c). A transverse section of an embryo at 4 pss is shown in (d). (e–g) Immunofluorescence staining ofWnt3(mVenus) BAC transgenic embryos for mVenus with antibodies to GFP at 3 pss (e), 4 pss (f) and 5 pss (g). (h) WISH analysis ofmNkd1mRNA at 3 pss. (i–k) X-gal staining ofmNkd1(lacZ) BAC transgenic embryos at 2 pss (i), 3 pss (j) and 4 pss (k). Open and closed arrowheads indicate not-expressed or expressed, respectively. (l) Schematic representation ofWnt3, showing a putative TCF-binding site located 75 bp upstream of the initiation codon, as well as ofWnt3(lacZ) andWnt3(lacZ-ΔTCF) constructs. (m) X-gal staining of aWnt3(lacZ) BAC transgenic embryo at 4 pss. (n,o) Results of an F0 assay forWnt3(lacZ) (n) andWnt3(lacZ-ΔTCF) (o) BACs. (p,q) Node explants fromWnt3(LacZ)BACtransgenic embryos were cultured without (p) or with (q) Wnt3A protein (0.8 μg ml−1). Note thatlacZexpression at the node was upregulated by Wnt3A protein. Scale bars, 50 μm. Figure 4: Asymmetric expression of Wnt3 and its regulation by Wnt signalling. ( a – d ) WISH analysis of Wnt3 expression at 2 pss ( a ), 3 pss ( b ) and 4 pss ( c ). A transverse section of an embryo at 4 pss is shown in ( d ). ( e – g ) Immunofluorescence staining of Wnt3 ( mVenus ) BAC transgenic embryos for mVenus with antibodies to GFP at 3 pss ( e ), 4 pss ( f ) and 5 pss ( g ). ( h ) WISH analysis of mNkd1 mRNA at 3 pss. ( i – k ) X-gal staining of mNkd1 ( lacZ ) BAC transgenic embryos at 2 pss ( i ), 3 pss ( j ) and 4 pss ( k ). Open and closed arrowheads indicate not-expressed or expressed, respectively. ( l ) Schematic representation of Wnt3 , showing a putative TCF-binding site located 75 bp upstream of the initiation codon, as well as of Wnt3 ( lacZ ) and Wnt3 ( lacZ- Δ TCF ) constructs. ( m ) X-gal staining of a Wnt3 ( lacZ ) BAC transgenic embryo at 4 pss. ( n , o ) Results of an F0 assay for Wnt3 ( lacZ ) ( n ) and Wnt3 ( lacZ- Δ TCF ) ( o ) BACs. ( p , q ) Node explants from Wnt3 ( LacZ ) BAC transgenic embryos were cultured without ( p ) or with ( q ) Wnt3A protein (0.8 μg ml −1 ). Note that lacZ expression at the node was upregulated by Wnt3A protein. Scale bars, 50 μm. Full size image The level of canonical Wnt activity was also found to be asymmetric around the node, consistent with previous observations [14] . Expression of mNkd1 , a gene that responds to Wnt signalling [15] , thus manifested L>R asymmetry around the node (1/6, 0/1, 10/10, 9/9 and 7/7 embryos showed asymmetric expression at 1, 2, 3, 4 or 5 pss, respectively) ( Fig. 4h ). The L–R asymmetry of Wnt activity was further confirmed by examination of embryos harbouring the mNkd1 ( lacZ ) BAC transgene, in which the coding sequence for β-galactosidase is intercalated into start site of mNkd1 . Staining of transgenic embryos with the β-galactosidase substrate X-gal (5-bromo-4-chloro-indolyl-β- D -galactopyranoside) revealed subtle asymmetry of lacZ expression at 2 pss (3/3 embryos)( Fig. 4i ) and marked asymmetry at 3 pss (2/2 embryos) ( Fig. 4j ) and 4 pss (5/5 embryos) ( Fig. 4k ). These results thus indicated that Wnt signalling activity becomes asymmetric slightly later than does expression of Cerl2 (late headfold stage to 1 pss) [16] . To examine the role of asymmetric Wnt signalling around the node in asymmetric expression of Cerl2 , we examined the effect of conditional deletion of the β-catenin gene by crossing β catenin flox/flox mice with ROSA CreERT2/+ , β catenin flox/+ mice [17] . Tamoxifen (5 mg per body in corn oil) was administered orally to the pregnant mice twice at embryonic day (E) 7.25 and E7.75 in order to activate the Cre recombinase [18] , and embryos were recovered at E8.5. Most of the conditional knockout embryos failed to manifest L<R asymmetry of Cerl2 expression at 4 pss (13/15 embryos) ( Fig. 5a–d ); Cerl2 expression was thus R=L (6/15 embryos) ( Fig. 5d ), bilaterally absent (7/15 embryos) ( Fig. 5b ), or L<R (2/15 embryos) ( Fig. 5c ). To determine whether the variability in the pattern of Cerl2 expression in the mutant embryos was because of variable effects of tamoxifen, we simultaneously examined individual embryos for mNkd1 and Cerl2 expression. In control embryos, mNkd1 expression was apparent around the primitive streak ( Fig. 5e ) and Cerl2 expression was asymmetric ( Fig. 5f ). In the mutant embryos that had lost mNkd1 expression, however, R>L asymmetry of Cerl2 expression was impaired showing at most only subtle R>L asymmetry around the node ( Fig. 5g ). We also examined individual embryos for β catenin protein and Cerl2 mRNA ( Supplementary Fig. S5e –h). In embryos in which β-catenin was severely lost ( Supplementary Fig. S5g ,h), asymmetry of Cerl2 mRNA was impaired. The position of the basal body remained posterior in the pit cells of the node in the conditional knockout embryos ( Supplementary Fig. S5a –d). Wnt signalling acts to reduce the level of Cerl2 mRNA as incubation of node explants from late headfold stage embryos with excess Wnt3A protein resulted in downregulation of Cerl2 mRNA ( Supplementary Fig. S5i ,j). These various observations suggested that Wnt signalling might amplify an initial asymmetry in Cerl2 expression established by nodal flow. 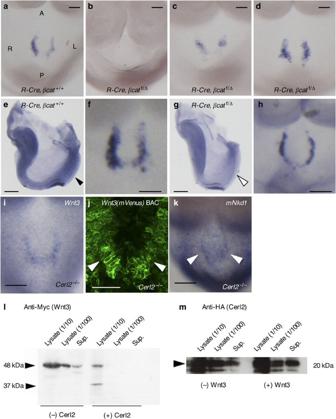Figure 5: Wnt signalling is required for asymmetry ofCerl2mRNA around the node. (a–d) WISH analysis ofCerl2expression with exon probe inROSACreERT2, βcatenin+/+(a) andROSACreERT2, βcateninflox/flox(b–d) embryos at E8.5 after exposure to tamoxifen during gestation. The conditional knockout embryos showed no (b), slightly asymmetric (c), or symmetric (d) expression ofCerl2. (e–h) Simultaneous detection ofmNkd1andCerl2expression inROSACreERT2, βcatenin+/+(e,f) andROSACreERT2, βcateninflox/flox(g,h) embryos at E8.5 after exposure to tamoxifen during gestation. Closed and open arrowheads indicatemNkd1expression at the primitive streak and the absence of such expression, respectively. The loss ofmNkd1expression was associated with only a slight asymmetry ofCerl2mRNA around the node. (i) WISH analysis ofWnt3mRNA in aCerl2−/−embryo at 4 pss. (j) Immunofluorescence staining of mVenus with antibodies to GFP in aCerl2−/−embryo harbouring theWnt3(mVenus) BAC transgene at 4 pss. (k) WISH analysis ofmNkd1expression in aCerl2−/−embryo at 4 pss. (l) Immunoblot analysis with antibodies to Myc for lysates (1/10 and 1/100 dilutions) and culture supernatants (Sup.) of Cos7 cells transfected with an expression vector for Wnt3-5 × Myc (48 kDa) with or without a vector for Cerl2-HA. (m) Immunoblot analysis with antibodies to HA for lysates (1/10 and 1/100 dilutions) and culture supernatants (Sup.) of Cos7 cells transfected with an expression vector for Cerl2-HA (20 kDa) with or without a vector for Wnt3-5 × Myc. See alsoSupplementary Fig. S4. Scale bars: 50 μm (a–d,f,h,i–k), Scale bars, 50 μm(for example). Figure 5: Wnt signalling is required for asymmetry of Cerl2 mRNA around the node. ( a – d ) WISH analysis of Cerl2 expression with exon probe in ROSA CreERT2 , β catenin +/+ ( a ) and ROSA CreERT2 , β catenin flox/flox ( b – d ) embryos at E8.5 after exposure to tamoxifen during gestation. The conditional knockout embryos showed no ( b ), slightly asymmetric ( c ), or symmetric ( d ) expression of Cerl2 . ( e – h ) Simultaneous detection of mNkd1 and Cerl2 expression in ROSA CreERT2 , β catenin +/+ ( e , f ) and ROSA CreERT2 , β catenin flox/flox ( g , h ) embryos at E8.5 after exposure to tamoxifen during gestation. Closed and open arrowheads indicate mNkd1 expression at the primitive streak and the absence of such expression, respectively. The loss of mNkd1 expression was associated with only a slight asymmetry of Cerl2 mRNA around the node. ( i ) WISH analysis of Wnt3 mRNA in a Cerl2 −/− embryo at 4 pss. ( j ) Immunofluorescence staining of mVenus with antibodies to GFP in a Cerl2 −/− embryo harbouring the Wnt3 ( mVenus ) BAC transgene at 4 pss. ( k ) WISH analysis of mNkd1 expression in a Cerl2 −/− embryo at 4 pss. ( l ) Immunoblot analysis with antibodies to Myc for lysates (1/10 and 1/100 dilutions) and culture supernatants (Sup.) of Cos7 cells transfected with an expression vector for Wnt3-5 × Myc (48 kDa) with or without a vector for Cerl2-HA. ( m ) Immunoblot analysis with antibodies to HA for lysates (1/10 and 1/100 dilutions) and culture supernatants (Sup.) of Cos7 cells transfected with an expression vector for Cerl2-HA (20 kDa) with or without a vector for Wnt3-5 × Myc. See also Supplementary Fig. S4 . Scale bars: 50 μm ( a – d , f , h , i – k ), Scale bars, 50 μm(for example). Full size image Wnt3 asymmetry is controlled by Cerl2 and Wnt signalling Examination of the nucleotide sequence of mouse Wnt3 revealed a consensus binding sequence (ACTTTGT) for the transcription factor TCF that is located 75 bp upstream of the initial codon ( Fig. 4l ) and that is conserved among all mammals examined and chick. We examined the role of this putative TCF-binding site with the use of the Wnt3 ( lacZ ) BAC transgene, in which the first exon of Wnt3 is replaced by lacZ . Embryos harbouring this transgene showed L>R asymmetric expression of lacZ around the node at 3 pss (5/5 embryos) ( Fig. 4m ). However, mice harbouring the Wnt3 ( lacZ- Δ TCF ) BAC transgene, in which the putative TCF-binding sequence is mutated, showed bilateral and downregulated expression of lacZ (6/6 embryos) ( Fig. 4o ). Furthermore, incubation of embryos harbouring Wnt3 ( lacZ ) BAC transgene with Wnt3A-stimulated lacZ expression ( Fig. 4p ). These results indicated that Wnt3 expression is upregulated on the left side of the node by Wnt signalling. Given that Wnt proteins are potential targets of Cer/DAN family proteins [19] , [20] , we also examined whether Wnt3 expression and Wnt activity are regulated by Cerl2. Expression of Wnt3 , which is L>R asymmetric in the wild-type embryo, was symmetric in a Cerl2 –/– mutant (2/2, 2/2 and 4/4 embryos at 2, 3 or 4 pss, respectively) ( Fig. 5i ). Expression of the Wnt3 ( mVenus ) BAC transgene and mNkd1 was also symmetric in the Cerl2 mutant (2/2 embryos at 3 pss, 3/3 embryos at 4 pss) ( Fig. 5j ), suggesting that L>R asymmetry of Wnt3 expression and Wnt activity requires Cerl2. Although proteins of the Cer/DAN family have been suggested to inhibit Wnt signalling, their precise action has remained unknown. To examine possible interaction between Wnt3 and Cerl2, we introduced an expression vector for Myc epitope–tagged Wnt3, with or without an expression vector for Cerl2, into Cos7 cells. The amount of Wnt3-5 × Myc in both culture supernatants and cell lysates was markedly reduced for cells coexpressing ectopic Cerl2 ( Fig. 5l ). This reduction appeared to result, at least in part, from protein degradation, given that an immunoreactive protein with a smaller molecular size (~37 versus 48 kDa) was detected only in lysates prepared from cells coexpressing Cerl2 ( Fig. 5l ). On the other hand, the amount of hemagglutinin epitope (HA)–tagged Cerl2 was not affected by coexpression of ectopic Wnt3 ( Fig. 5m ). In the mouse embryo, Wnt3a (a gene highly related to Wnt3 , with the encoded proteins showing 84.9% amino-acid sequence identity) is also expressed around the node and primitive streak. The amount of ectopic Wnt3A in lysates and culture supernatants of Cos7 cells or Xenopus oocytes was also reduced by coexpression of Cerl2 ( Supplementary Fig. S5k ,l). These results suggested that asymmetric (L<R) degradation of Wnt3 and Wnt3A induced by Cerl2 in mouse embryos renders Wnt signalling activity asymmetric (L>R). The L>R asymmetric expression of Wnt3 thus requires canonical Wnt signalling, which is preferentially inhibited on the right side by Cerl2. Both the flow and Wnt signals promote decay of Cerl2 mRNA The abundance of Cerl2 mRNA is regulated at a post-transcriptional level in a manner-dependent on nodal flow and Wnt signals. To dissect the actions of the flow signal and Wnt signal separately, we first incubated embryos that are isolated at early head fold stage with BIO (6-bromo-indirubin-3′-oxime, an activator of canonical Wnt signalling) in the absence or presence of actinomycin D. Incubation of embryos with BIO alone for 12 h (which resulted in upregulation of mNkd1 expression but did not affect Nodal and Gdf1 expression: Supplementary Fig. S6a –d, m, n) reduced the level of Cerl2 mRNA and abolished its L<R asymmetry ( Fig. 6a ; 3/3 embryos). BIO also showed similar effects in the presence of actinomycin D ( Fig. 6c ; 7/7 embryos) while it did not affect the level of Brachyury mRNA ( Supplementary Fig. S6i ,j), suggesting that Wnt signalling regulates Cerl2 expression at a post-transcriptional level. We next incubated early head fold stage embryos with IWR-1 (a synthetic inhibitor of canonical Wnt signalling) for 12 h, which did not affect Nodal and Gdf1 expression ( Supplementary Fig. S6e –h) but abolished mNkd1 expression ( Supplementary Fig. S6k ,l). Such treatment reduced the extent of but did not abolish the L<R asymmetry of Cerl2 ( sGFP ) mRNA in embryos harbouring the Cerl2 ( sGFP ) BAC transgene ( Fig. 6e ; 3/3 embryos). In contrast, embryos harbouring the Cerl2 ( sGFP- Δ 3 ′ -UTR ) BAC transgene failed to show asymmetry of Cerl2 mRNA in the presence of IWR-1 ( Fig. 6f ), suggesting that the flow signal acts on Cerl2 mRNA via its 3′-UTR. Together, these results thus indicated that both the flow signal and Wnt signal promote the decay of Cerl2 mRNA. 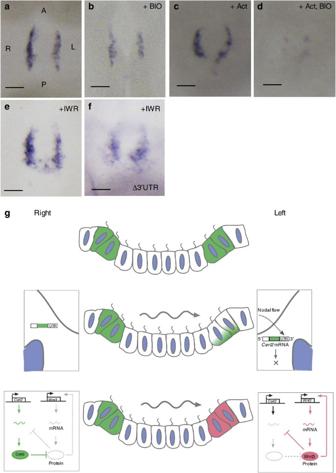Figure 6: Both Flow and Wnt Signals Promote Decay ofCerl2mRNA. (a,b) WISH analysis ofCerl2mRNA (exon probe) in embryos isolated at EHF and incubated for 12 h in the absence (a) or presence (b) of 75 μM BIO. (c,d) WISH analysis ofCerl2mRNA (exon probe) in embryos isolated at EHF and incubated for 12 h with 1 μg ml−1actinomycin D (ACT) in the absence (c) or presence (d) of 75 μM BIO. (e,f) WISH analysis ofCerl2(sGFP) mRNA in embryos harbouring theCerl2(sGFP) BAC (e) orCerl2(sGFP-Δ3′UTR) BAC (f) transgenes that were isolated at EHF and incubated for 12 h with 60 μM IWR-1. (g) Summary of the mechanism that converts the signal transmitted by nodal flow into robust asymmetry ofCerl2expression. See the text for detail. Scale bars, 50 μm. Figure 6: Both Flow and Wnt Signals Promote Decay of Cerl2 mRNA. ( a , b ) WISH analysis of Cerl2 mRNA (exon probe) in embryos isolated at EHF and incubated for 12 h in the absence ( a ) or presence ( b ) of 75 μM BIO. ( c , d ) WISH analysis of Cerl2 mRNA (exon probe) in embryos isolated at EHF and incubated for 12 h with 1 μg ml −1 actinomycin D (ACT) in the absence ( c ) or presence ( d ) of 75 μM BIO. ( e , f ) WISH analysis of Cerl2 ( sGFP ) mRNA in embryos harbouring the Cerl2 ( sGFP ) BAC ( e ) or Cerl2 ( sGFP- Δ 3 ′ UTR ) BAC ( f ) transgenes that were isolated at EHF and incubated for 12 h with 60 μM IWR-1. ( g ) Summary of the mechanism that converts the signal transmitted by nodal flow into robust asymmetry of Cerl2 expression. See the text for detail. Scale bars, 50 μm. Full size image Role of interlinked feedback loops involving Cerl2 and Wnt Cerl2 and Wnt contribute to interlinked feedback loops that include a double-negative loop between Cerl2 and Wnt as well as the self-activating loop of Wnt. Flow provides an initial L–R bias in Cerl2 expression, which is subsequently amplified by the Wnt-Cerl2 feedback loops ( Fig. 7a ). To reveal the dynamic properties of these interlinked feedback loops and to examine their role in establishment of robust asymmetry of gene expression, we constructed a mathematical model ( Fig. 7a , see Supplementary Experimental Procedures; Supplementary Figs S7,S8 ). The dynamics of gene activity on the left and right sides of the node were considered separately by assignment of different inputs of the flow signal to the left and right sides; two ordinary differential equation systems (right and left systems) were thus set, with only the left system receiving the flow signal. 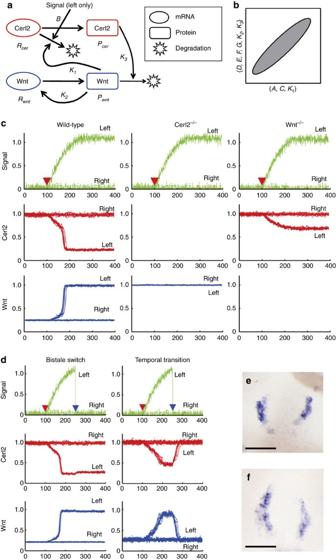Figure 7: Mathematical model and numerical analysis of L–R asymmetry of gene expression. (a) Diagram showing the regulation ofCerl2andWntexpression. (b) Schematic representation of conditions of parameters. SeeSupplementary Experimental Proceduresfor details. (c) Examples of the dynamics of gene activities obtained by computer simulation. The vertical axis represents the level of the signal (top),Pcer(middle) orPwnt(bottom). The horizontal axis is time. The results of 10 calculations are shown. Simulations are shown for wild-type embryos,Cerl2−/−embryos (Rcerfixed to 0), andWnt−/−embryos (Rwntfixed to 0). (d) Dynamics of gene activities under conditions of perturbation of the signal. The signal is shut down in the left system att′=250. Results of 10 calculations are shown. The axes are as in (c). Simulations are for systems with the mechanisms ‘bistable switch’ or ‘temporal transition to asymmetric state.’ (e,f) Whole-mount FISH analysis ofCerl2expression (exon probe) in embryos isolated at 1 pss and cultured for 4 h in the absence (e) or presence (f) of 1% methyl cellulose. Scale bars: 50 μm. Figure 7: Mathematical model and numerical analysis of L–R asymmetry of gene expression. ( a ) Diagram showing the regulation of Cerl2 and Wnt expression. ( b ) Schematic representation of conditions of parameters. See Supplementary Experimental Procedures for details. ( c ) Examples of the dynamics of gene activities obtained by computer simulation. The vertical axis represents the level of the signal (top), P cer (middle) or P wnt (bottom). The horizontal axis is time. The results of 10 calculations are shown. Simulations are shown for wild-type embryos, Cerl2 −/− embryos ( R cer fixed to 0), and Wnt −/− embryos ( R wnt fixed to 0). ( d ) Dynamics of gene activities under conditions of perturbation of the signal. The signal is shut down in the left system at t ′=250. Results of 10 calculations are shown. The axes are as in ( c ). Simulations are for systems with the mechanisms ‘bistable switch’ or ‘temporal transition to asymmetric state.’ ( e , f ) Whole-mount FISH analysis of Cerl2 expression (exon probe) in embryos isolated at 1 pss and cultured for 4 h in the absence ( e ) or presence ( f ) of 1% methyl cellulose. Scale bars: 50 μm. Full size image Analysis of the model by numerical simulation confirmed that it can reproduce the observed patterns of gene expression if appropriate values are assigned to the parameters ( Fig. 7c ). In the computer simulation for the wild-type embryo, a small-amplitude signal in the left system induces a large change in the expression of Cerl2 and Wnt and results in final L–R asymmetry. In the Cerl2 −/− embryo, however, Wnt expression remains bilaterally high. In a Wnt −/− embryo, Cerl2 expression is high on both sides, although there is a small L<R asymmetry. By calculating the dynamics of the model multiple times with randomly chosen parameter values, we examined the ability of each simulation to reproduce observed patterns of gene expression (see Supplementary Experimental Procedures). The distribution of parameter values in the set of successful simulations suggested important properties of parameters ( Fig. 7b ). The parameters are categorized into two groups in terms of their effects on dynamics, ( A , C , K 1 ) and ( D , E , F , G , K 2 , K 3 ). Increasing the values of the former group of parameters increases the level of Cerl2 expression at steady state, whereas increasing those of the latter group increases the level of Wnt expression. When values for the two groups of parameters are balanced (within the grey region in Fig. 7b ), the model can reproduce the observed gene expression patterns. From the numerical and mathematical analysis, we identified two essential mechanisms for asymmetric gene expression that depend on parameter values: ‘bistable switch’ and ‘temporal transition to asymmetric state’ ( Fig. 7d ). The role of the flow signal distinguishes these two mechanisms: In the former mechanism, after the flow signal induces a subtle decrease in the amount of Cerl2 mRNA on the left side, the interlinked feedback loops amplify the small asymmetry and stably lock the state of gene expression. Flow is thus not continuously required. In the latter mechanism, however, the flow signal is continuously required to generate and maintain the state of gene expression on the left. Parameter sensitivity analysis showed that the ‘bistable switch’ mechanism is observed in a much broader area than is ‘temporal transition to asymmetric state’ (see Supplementary Fig. S9 ). Given that nodal flow is maintained during the period of asymmetric gene expression in the mouse embryo, it was not possible to distinguish which of the two mechanisms (‘bistable switch’ or ‘temporal transition to asymmetric state’) operates in vivo . We addressed this issue experimentally by examining whether continuous flow is required for L–R asymmetric Cerl2 expression in embryos in culture. Embryos at 1 pss, which have received the temporal flow signal, were cultured for 4 h in the absence ( Fig. 7e ) or presence ( Fig. 7f ) of 1% methylcellulose. As reported previously [16] , 1% methylcellulose completely abolishes the flow (see Supplementary Fig. S10 ). These embryos treated with 1% methylcellulose still developed L<R asymmetric Cerl2 expression ( Fig. 7f ) suggesting that the flow is required only temporarily. We therefore conclude that the Wnt - Cerl2 regulatory circuit functions as a bistable switch that makes possible the generation of asymmetric gene expression even under unstable, noisy conditions. Our data suggest how the signal transmitted by nodal flow is converted into robust asymmetry of Cerl2 expression ( Fig. 6g ). Expression of Cerl2 is symmetric around the node before generation of fluid flow. The onset of asymmetric fluid flow triggers the degradation of Cerl2 mRNA in a manner dependent on it 3′-UTR in the apical region of crown cells on the left side of the node. Inhibition of a Wnt3-positive feedback loop by Cerl2 is then relieved on the left side, resulting in an increase in the amount of Wnt3. In turn, the Wnt signal further reduces the amount of Cerl2 mRNA on the left. These interlinked feedback loops including Wnt signalling and Cerl2 thus transform the small asymmetry in Cerl2 mRNA induced by nodal flow into a robust asymmetry. Post-transcriptional regulation of gene expression at the level of mRNA decay has been shown to operate in various cell types [21] . The largest and best studied group of cis-acting sequences that determine mRNA instability are AU-rich elements (AREs). The canonical ARE contains one or multiple copies of the sequence AUUUA in a U-rich region of the 3′-UTR. Several proteins that bind to the ARE have been identified, most of which destabilize ARE-containing mRNAs. Although Cerl2 mRNA contains ARE-like sequences in its 3′-UTR, the relevance of these sequences is unknown. Our results suggest that both the initial flow-derived signal and subsequent Wnt-mediated signalling promote degradation of Cerl2 mRNA on the left side of the node ( Fig. 6g ). The absence of Cerl2 mRNA in the apical region of left crown cells in wild-type embryos as well as the accumulation of Cerl2 mRNA in this region in a mutant ( iv/iv ) lacking nodal flow suggest that the mRNA is degraded at the apical side of left crown cells in response to the flow. Given that the Ca 2+ channels Pkd2 and Pkd1l1 are required for flow detection [22] , [23] , [24] , [25] , Ca 2+ signalling may contribute to the degradation of Cerl2 mRNA. How does Wnt signalling regulate Cerl2 mRNA stability? In addition to regulation of transcription, β-catenin also regulates RNA stability [26] , [27] . For example, β-catenin, together with the RNA-binding protein HuR, recognizes a specific RNA motif in the 3′-UTR of COX2 mRNA in colon cancer cells [28] . Similarly, AU-rich motifs in the 3′-UTR of Cerl2 mRNA may be a target of β-catenin. Alternatively, β-catenin may indirectly promote the decay of Cerl2 mRNA via transcriptional activation of a gene for an RNA-binding protein. Noise-resistant mechanisms are essential for development to proceed with high accuracy. Indeed, interlinked signalling feedback loops involving BMP, GREM1 (a BMP inhibitor), fibroblast growth factor and sonic hedgehog constitute a self-regulatory network that underlies accurate development of the mouse distal limb [29] . The interlinked feedback loops connecting Cerl2 and Wnt identified in the present study are able to convert the initial small bias in Cerl2 mRNA distribution conferred by nodal flow into a robust asymmetry, and they behave as a noise-resistant network. This finding is consistent with previous theoretical modelling suggesting that multiple interlinked feedback loops, rather than a single-positive feedback loop, can produce decisive outputs in a manner resistant to noise in the upstream signalling system [30] . Nodal flow is one of several processes that fluctuate during L–R decision making, with the velocity of the flow having been found to fluctuate within a short-time period (see Supplementary Fig. S11 ). We previously showed that L–R asymmetric expression of Nodal in the LPM is established by a SELI system [8] . A SELI system consisting of Nodal and Lefty thus generates robust L–R asymmetry in LPM by relying on the node-derived asymmetric signal. The network of Wnt-Cerl2 interlinked feedback loops identified in the present study is responsible for generation of L–R asymmetry at the node, which is then made use of by the SELI system in LPM. The operation of both systems thus ensures that the initial small bias provided by nodal flow is gradually amplified and finally converted to exclusive asymmetry, such as asymmetric Nodal expression in LPM. It remains unknown whether the Wnt-Cerl2 interlinked feedback loops are conserved among vertebrates. Such a system has not yet been found to operate around the ventral node or organizer of other vertebrates. However, several Wnt genes are expressed around the organizer in other organisms [31] , and Cerl2 homologues, including Charon in zebrafish [32] and Coco in Xenopus [33] , are also expressed near the organizer, suggesting that similar interlinked feedback loops may indeed operate in other vertebrates. Alternatively, the interlinked feedback loops may be specific to mammals, which may be one of the reasons why L–R patterning of mammals, such as mouse and human, is highly accurate (incidence of spontaneous reversal of heart asymmetry in mammals is lower than that in other vertebrates [34] ). Quantitative analysis of mRNA abundance by FISH Whole-mount FISH was performed as previously described [35] . The method for FISH was similar to that described for zebrafish embryos [36] , with the exceptions that a tetrahydroborate step was added to reduce background fluorescence before hybridization of RNA probes and that probes labelled with dinitrophenol were used instead of those labelled with fluorescein isothiocyanate. The linearity of the FISH signal was tested as described in Supplementary Experimental Procedures. Two and six different intron probes were used for Nodal and Cerl2 mRNAs, respectively. These probes were located at positions 1,151–1,590 bp (relative to the translation start site) and 2,301–2,800 bp for Nodal , and at positions 360–578, 1,179–1,476, 1,866–2,135, 2,448–2,609, 5,266–5,403, and 5,954–6,156 bp for Cerl2 . To stain the apical membrane of crown cells after FISH, we soaked embryos in phosphate-buffered saline containing VivrantDiI (Invitrogen) at a 1/100 dilution for 1 min. To simultaneously detect β catenin protein and Cerl2 mRNA in the node, we performed FISH followed by the standard immunostaining procedure with an anti-β catenin antibody (Millipore). Immunofluorescence staining The level of pSmad2 was examined with specific antibodies as previously described [6] . For quantitation of the pSmad2 signal, fluorescence images of the node were processed by ImageJ software. The level of background fluorescence was estimated by averaging background values at four points of each image and was subtracted from the fluorescence in crown cells. Areas of fluorescence were then marked manually, and fluorescence values were calculated automatically. Immunofluorescence staining was also performed with antibodies to β-galactosidase (Abcam), to GFP(MBL), to Odf2 (gifted by Dr S Tsukita) and to E-cadherin (TAKARA). Generation of transgenic mice Wnt3 BAC transgenes were constructed from the mouse Wnt3 BAC clone RP23-31D10. In the Wnt3 ( mVenus ) BAC, the first exon of Wnt3 was replaced by the coding sequence for membrane-localized Venus, which consists of cDNA for Venus and for the NH 2 -terminal sequence of neuromodulin (nucleotides 679–738) from pECFP-mem (BD Biosciences). In the Wnt3 ( lacZ ) BAC, the first exon of Wnt3 was replaced by the coding sequence for LacZ. In the Wnt3 ( lacZ- Δ TCF ) BAC, the putative TCF-binding site (ACTTTGT) located 75 bp upstream of the initiation codon was replaced with the sequence ACGGGGT. The mNkd1 BAC transgene was constructed from the mouse mNkd1 BAC clone RP23-258C7. In the mNkd1 ( lacZ ) BAC, the first exon of mNkd1 was replaced by the coding sequence for LacZ. The Cerl2 BAC transgene was constructed from the mouse Cerl2 BAC clone RP23-421H21. In the Cerl2 ( lacZ ) BAC, the first exon of Cerl2 was replaced by the coding sequence for LacZ and the polyadenylation signal sequence (250 bp) of SV40. In the Cerl2 ( sGFP ) BAC, a 300-bp sequence coding for a portion of EGFP was inserted in-frame into the Sma I site located in exon 2 of Cerl2 . In the Cerl2 ( sGFP- Δ 5 ′ -UTR ) BAC, the 5′-UTR of Cerl2 was replaced by the 5′-UTR of mouse Hprt . In the Cerl2 ( sGFP- Δ intron ) BAC, intron 1 of Cerl2 had been excised. In the Cerl2 ( sGFP- Δ 3 ′ -UTR ) BAC, the 3′-UTR of Cerl2 was replaced by the polyadenylation signal sequence (250 bp) of SV40. All transgenic mice were established as previously described [37] . In some cases (when indicated as F0 assay), transgenic embryos were directly examined before establishing stable transgenic lines. After injection of each constructs into fertilized eggs, eggs were transferred pseudo pregnant mother again. At around E8.5, embryos were recovered and processed by LacZ staining. Recombinant BAC clones were constructed with the use of the highly efficient BAC-based recombination system for Escherichia coli [38] . BAC DNA was prepared for microinjection as previously described [39] . The study was approved by the animal experimentation committee of Osaka University. Interaction of Cerl2 and Wnt Wnt3 cDNA containing the entire open-reading frame (ORF) was cloned by the PCR from RNA prepared from E8.25 mouse embryos and was inserted into the expression vector pBOS-EX. A DNA sequence encoding four tandem repeats of the Myc epitope tag was then inserted at the 3′-end of the Wnt3 ORF. A double-stranded oligonucleotide corresponding to three tandem repeats of the HA tag was inserted in front of the stop codon of the Cerl2 ORF in pBOS-EX. The Wnt3a ORF was also subcloned into pBOS-EX. Cos7 cells were transferred to 24-well plates and cultured to subconfluence in Dulbecco’s modified Eagle’s medium (DMEM) supplemented with 10% foetal bovine serum. The medium was replaced with OPTI-MEM (Invitrogen) immediately before lipofection. The expression vectors for Wnt3-5 × Myc, Wnt3A and Cerl2-3 × HA were introduced into the cells with the use of Lipofectamine LTX (Invitrogen). Culture supernatants were collected and cell lysates were prepared for immunoblot analysis after lipofection for 2 days. The ORFs for Wnt3A and Cerl2-3 × HA were also subcloned into pSP64T [40] , and capped synthetic mRNAs were transcribed with the use of an mMessage mMachine kit (Ambion). Xenopus oocytes were injected with 50 ng of each mRNA and then cultured for 3 days at 20 °C in modified Barth’s solution. Conditioned medium was then collected and cell lysates were prepared for immunoblot analysis. Immunoblot analysis was performed with antibodies to Myc (Santa Cruz), to HA and to Wnt3A (Abcam). Embryo culture All embryonic culture were performed under 5% CO2, 75% rat serum and 25% DMEM (Invitrogen). Embryos were rotated in a 50-ml falcon tube. Concentrations of each reagent are as following. Actinomycin D: 1 μg ml −1 , BIO: 75 μM, IWR: 60 μM. Node explants were cultured under the same condition without rotation after dissection. Concentrations of Wnt3A protein (R&D systems) was 0.8 μg ml −1 . Other experimental procedures Quantitative FISH analysis, quantitation of nodal flow velocity and mathematical modelling are described in detail in Supplementary Experimental Procedures. How to cite this article: Nakamura, T. et al . Fluid flow and interlinked feedback loops establish left–right asymmetric decay of Cerl2 mRNA. Nat. Commun. 3:1322 doi: 10.1038/ncomms2319 (2012).